Impermeable barrier films and protective coatings based on reduced graphene oxide Flexible barrier films preventing permeation of gases and moistures are important for many industries ranging from food to medical and from chemical to electronic. From this perspective, graphene has recently attracted particular interest because its defect-free monolayers are impermeable to all atoms and molecules. However, it has been proved to be challenging to develop large-area defectless graphene films suitable for industrial use. Here we report barrier properties of multilayer graphitic films made by gentle chemical reduction of graphene oxide laminates with hydroiodic and ascorbic acids. They are found to be highly impermeable to all gases, liquids and aggressive chemicals including, for example, hydrofluoric acid. The exceptional barrier properties are attributed to a high degree of graphitization of the laminates and little structural damage during reduction. This work indicates a close prospect of graphene-based flexible and inert barriers and protective coatings, which can be of interest for numerous applications. Membranes made from graphene and its chemical derivative called graphene oxide [1] , [2] , [3] (GO) show a range of unique barrier properties [4] , [5] , [6] , [7] , [8] . Defect-free monolayer graphene is impermeable to all gases and liquids [4] and, similar to graphite, shows high chemical and thermal stability with little toxicity. These characteristics are believed to provide graphene with a competitive edge over the existing barrier materials [9] . Unfortunately, prospects of using graphene as a protective coating are hampered by difficulties of growing large-area defect-free films. For example, it is shown that graphene films grown by chemical vapour deposition (CVD) possess many defects and grain boundaries and do not protect copper against oxidation but, to the contrary, speed up its corrosion [10] . A potential solution to this problem is the use of graphene-based multilayers [11] , [12] , [13] . In this respect, GO is particularly attractive because multilayer films can be produced easily and relatively cheaply by depositing GO solutions on various substrates by spraying, and dip- or rod-coating, and so on. The resulting GO laminates are shown to exhibit highly unusual permeation properties [5] , [6] , [7] , [8] . In the dry state, they are impermeable even for helium but, under humid conditions, provide no barrier for water vapour [5] . If immersed in water, the laminates act as molecular sieves allowing transport of small ions and blocking large ones [6] . Although such unique and contrasting properties may be useful for certain applications, many others need flexible barrier films with little oxygen and moisture permeation. The required rates are typically <0.1 g of water per m 2 per day and down to 10 −6 g m −2 per day in the case of flexible organic electronics [9] , [14] . Achieving these ultra-low rates for the case of flexible coatings is extremely challenging [14] . For comparison, the commonly used metallized polyethylene terephthalate (PET) films (40–50 nm Al on 12 μm PET further covered with a 75-μm low-density polyethylene) allow water permeation rates of ~0.5 g m −2 per day [15] . In this report, we explore the possibility of enhancing the barrier properties of GO laminates by using the fact that molecular permeation through them occurs along interlayer capillaries of ≈10 Å in width [5] , [6] . This distance can be decreased using chemical reduction and approaches 3.4 Å in bulk graphite. If no significant structural damage is induced by the process, it is reasonable to expect much improved barrier properties for reduced GO laminates. Considerable efforts have recently been made to utilize multilayer graphene-based films (thermally reduced GO (T-RGO) [11] , [12] , CVD graphene [13] and graphene-based composites [9] ) as ultra-barriers for organic electronics and as oxidation-resistant and anticorrosion coatings [9] , [16] , [17] , [18] , [19] , [20] , [21] , [22] . However, T-RGO membranes are extremely fragile and contain many structural defects, which results in notable water permeation [5] , [9] . A high density of defects in CVD graphene also limits its possible uses [9] , [10] . Similarly, GO-polymer composites have so far exhibited gas permeability too high to consider them for realistic applications [9] . To increase the quality of GO-based coatings, it is essential to decrease the number of defects formed during the reduction process [23] , [24] , [25] , [26] , [27] , [28] (see Supplementary Fig. 1 and Supplementary Note 1 ). Recent studies show that the use of hydroiodic (HI) acid as a reducing agent results in RGO’s quality being much higher than that provided by other reduction techniques, in terms of electrical and mechanical properties [25] , [27] , [29] . The HI reduction leaves fewer structural defects and little deformation so that the mechanical strength increases, becoming even higher than that for initial GO laminates that are known to be already exceptionally strong [1] . Another interesting reducing agent is ascorbic acid, that is, vitamin C (VC) [26] , [28] . It shows not only good reducing characteristics but stands out as environment friendly and nontoxic, which may be a critical factor in certain applications. Both reducing agents are believed to convert most of the functional groups attached to graphene into H 2 O, which results in little structural damage of graphene sheets during reduction [25] , [26] , [27] , [28] , [29] . In this contribution, we report permeation properties of GO laminates reduced using HI and VC. Both free-standing membranes and thin coatings on various substrates have been examined. Such RGO films are found to provide high-quality barriers that block all gases and liquids. In particular, if GO laminates are reduced in HI, no permeation of hydrogen and moisture could be detected for films as thin as 30 nm, which remain optically transparent. The films thicker than 100 nm exhibit no detectable permeation with respect to all tested gases and liquids. Furthermore, the RGO laminates are found to be impermeable to strong chemicals and salt solutions. These exceptional properties open a practical route towards graphene-based chemical-resistant and anticorrosion paints and coatings. 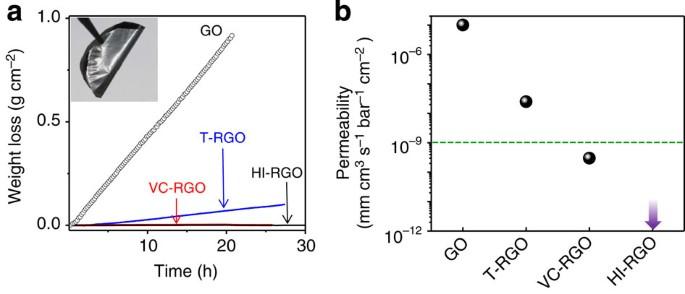Figure 1: Water permeation through free-standing multilayer graphene membranes. (a) Water loss from a container sealed with GO and RGO membranes with a diameter of ≈2 cm (thicknessd≈0.5 μm). For GO, the loss is the same as through an open aperture and limited by water evaporation. Inset: photo of an HI-RGO membrane (diameter ≈2 cm). (b) Permeability of various RGO membranes with respect to moisture. The arrow indicates our detection limit. Permeability of pristine GO is taken from ref.5. Green line: water permeability for the industrial-standard barrier films estimated using data of ref.30for 30 nm Al on PET. Permeation properties of free-standing RGO membranes Figure 1a shows examples of water permeation measurements through GO and RGO membranes. In agreement with the previous reports [5] , [6] , non-reduced membranes were found to be impermeable to all gases, except for H 2 O that evaporated with little resistance. After thermal reduction, the same membranes exhibited ~10 times slower water loss but became fragile. Permeation rates for three different T-RGO samples were measured and varied by a factor of 2. In contrast, GO membranes reduced in VC (VC-RGO) exhibited a decrease by 5 orders of magnitude in water transmission rates with respect to pristine GO laminates ( Fig. 1b ) with little (<20%) variation for six studied samples. HI-reduced GO membranes (HI-RGO; more than 10 samples) provided even a better barrier such that water permeation became undetectable within our best accuracy of ≈0.1 mg per week. This sets an upper limit for moisture permeation through HI-RGO films as 10 −2 g m −2 per day and ~10 −11 mm g s −1 bar −1 cm −2 (see Fig. 1b ). Despite being only the limit for our detection technique, this value is already nearly two orders of magnitude lower than water transparency for the industry-standard barrier films (aluminized PET) [30] . Note that the HI-RGO membranes were impermeable under both liquid and vapour conditions, with the former studied by using the same container but turned upside down so that liquid water was in direct contact with the membranes (See methods). As a crosscheck, we also performed measurements for several organic solvents such as acetone, methanol, ethanol and propanol and found no detectable permeation. Figure 1: Water permeation through free-standing multilayer graphene membranes. ( a ) Water loss from a container sealed with GO and RGO membranes with a diameter of ≈2 cm (thickness d ≈0.5 μm). For GO, the loss is the same as through an open aperture and limited by water evaporation. Inset: photo of an HI-RGO membrane (diameter ≈2 cm). ( b ) Permeability of various RGO membranes with respect to moisture. The arrow indicates our detection limit. Permeability of pristine GO is taken from ref. 5 . Green line: water permeability for the industrial-standard barrier films estimated using data of ref. 30 for 30 nm Al on PET. Full size image Permeation properties of RGO-coated PET It is more practical to use RGO not as free-standing membranes but as thin coatings on top of other materials. To evaluate barrier properties of such coatings, we have employed standard PET films (12-μm thick) as a support. 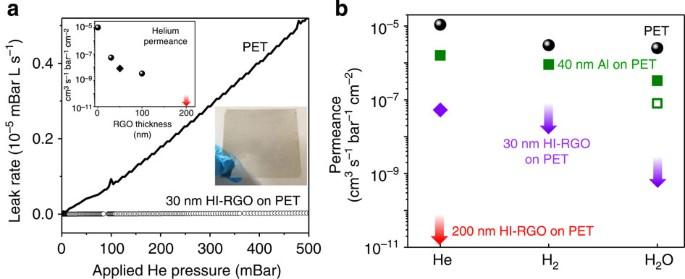Figure 2: Permeation through RGO barrier coatings. (a) He-leak measurements for a bare PET film (12 μm) and the same film coated with 30 nm of HI-RGO (normalized per cm2). The latter film is shown in the lower inset and exhibits an optical transparency of ≈35%. The transparency is reduced to 7% for 100-nm-thick RGO, and coatings thicker than 200 nm are opaque. Upper inset: He permeance (permeability divided byd) as a function of HI-RGO thicknessd(circles). The diamond symbol is for VC-RGO coating (d≈50 nm). (b) Barrier properties of bare PET, HI-RGO on PET and aluminized PET with respect to He, H2and H2O. Bare PET films (circles) show permeance in agreement with literature values33. The solid green symbols are for a 40-nm-thick aluminium film on PET (our measurements) and the open symbol is for a 30-nm Al on PET (ref.30). The violet and read arrows indicate our detection limits for 30 and 200 nm HI-RGO, respectively. Sample-to-sample variations for were less than 20%. Figure 2 shows an optical photo of the PET film covered with 30 nm of HI-RGO (See methods and Supplementary Fig. 2 ). Despite the much smaller thickness d than in the case of the RGO membranes discussed above, such optically transparent flexible barrier films show no detectable permeation of either hydrogen or water ( Fig. 2b ). Again, the moisture barrier is at least two orders of magnitude better than that provided by Al films of similar thickness. However, 30-nm-thick HI-RGO was still found to be slightly permeable to He, which can be attributed to occasional microscopic pinholes or structural defects in thin laminates that are made of randomly stacked graphene crystallites [5] , [6] , [7] , [8] . It requires HI-RGO films thicker than 100 nm to block He permeation completely, beyond the leak detection test that is the most sensitive method to check for potential leaks in high vacuum equipment (upper inset of Fig. 2a ). To assess the possible influence of humidity on He permeation [5] , we tested HI-RGO films in the presence of saturated water vapour and found no difference with respect to dry conditions. Furthermore, we carried out water permeation experiments at elevated temperatures of up to 45 °C and 100% humidity and found that the moisture barrier did not degrade. We have also tested a VC-RGO coating on PET and did not observe any significant difference with respect to HI-RGO. Importantly, chemically reduced GO exhibits strong adhesion to PET and, despite sub-micrometre thickness, withstands folding, stretching and moderate scratching, which allows normal handling procedures similar to Al-coated PET ( Supplementary Fig. 3 and Supplementary Note 2 ). Figure 2: Permeation through RGO barrier coatings. ( a ) He-leak measurements for a bare PET film (12 μm) and the same film coated with 30 nm of HI-RGO (normalized per cm 2 ). The latter film is shown in the lower inset and exhibits an optical transparency of ≈35%. The transparency is reduced to 7% for 100-nm-thick RGO, and coatings thicker than 200 nm are opaque. Upper inset: He permeance (permeability divided by d ) as a function of HI-RGO thickness d (circles). The diamond symbol is for VC-RGO coating ( d ≈50 nm). ( b ) Barrier properties of bare PET, HI-RGO on PET and aluminized PET with respect to He, H 2 and H 2 O. Bare PET films (circles) show permeance in agreement with literature values [33] . The solid green symbols are for a 40-nm-thick aluminium film on PET (our measurements) and the open symbol is for a 30-nm Al on PET (ref. 30 ). The violet and read arrows indicate our detection limits for 30 and 200 nm HI-RGO, respectively. Sample-to-sample variations for were less than 20%. Full size image Anticorrosion and chemical protection properties of RGO The discussed superior barrier properties of HI/VC-RGO laminates suggest their possible use as anticorrosion and chemical-resistant coatings [13] , [17] , [21] . To evaluate barrier properties with respect to salts and acids, we have used the measurement set-up described in ref. 6 . Briefly, two compartments of a U-shaped container were separated by a free-standing membrane and then filled, one with pure water and the other with a salt solution (concentrations varied from sub-Molar to full saturation). Salt diffusion was monitored by measuring its concentration in the pure water compartment by using ion chromatography and gravimetric analysis [6] . 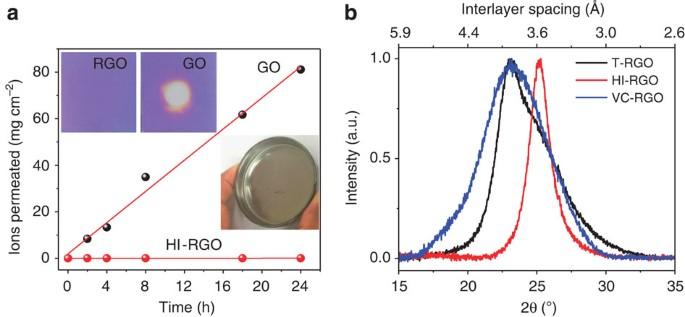Figure 3: Chemical protection by RGO. (a) Measurements of Cl-ion permeation through GO and HI-RGO membranes (d≈1 μm). Upper inset: right and left photos (1 cm × 1 cm) show the effect of HF on oxidized Si wafers protected by GO and RGO, respectively. SiO2is completely removed in the white centre region. Etching away of just 10 nm of SiO2would be visible as changes in the interference colour, which are absent in the left image. Bottom inset: glass petri dish lined with HI-RGO (≈1-μm thick). (b) X-ray diffraction for thermally, HI- and VC-reduced GO membranes. Figure 3a illustrates our results for the case of 1 M NaCl. Cl ions permeate rapidly through non-reduced GO membranes, in agreement with the earlier report [6] . However, within our experimental accuracy [6] , no salt permeation could be detected through either HI- or VC-RGO membranes. Figure 3: Chemical protection by RGO. ( a ) Measurements of Cl-ion permeation through GO and HI-RGO membranes ( d ≈1 μm). Upper inset: right and left photos (1 cm × 1 cm) show the effect of HF on oxidized Si wafers protected by GO and RGO, respectively. SiO 2 is completely removed in the white centre region. Etching away of just 10 nm of SiO 2 would be visible as changes in the interference colour, which are absent in the left image. Bottom inset: glass petri dish lined with HI-RGO (≈1-μm thick). ( b ) X-ray diffraction for thermally, HI- and VC-reduced GO membranes. Full size image To further illustrate anticorrosion properties of our graphitic laminates, we have tested their protection against HF, one of the most corrosive acids. The upper insets of Fig. 3a show the effect of HF on oxidized Si wafers (300 nm of SiO 2 ), which were protected with 0.5-μm-thick films of GO and VC-RGO. A drop of concentrated HF was placed on top of the coatings and continuously maintained for several hours. Then the coating was peeled off to assess damages. As evident from Fig. 3a , HF permeated through the GO film, as expected [6] , and etched through the entire thickness of the SiO 2 layer. On the other hand, the RGO film fully protected the wafer against HF, and no sign of SiO 2 etching could be detected within our accuracy of better than 10 nm. Similar acid drop tests were carried out for RGO coatings on top of various metals, including Cu and Ni. The latter foils were exposed to nitric and hydrochloric acids in different concentrations (0.1–10 M) but no degradation of the surface could be observed after several days of exposure. Furthermore, VC-RGO-coated Ni and steel foils were immersed in saturated iron chloride and sodium chloride solutions for many days and, again, no degradation could be detected. Finally, we covered glass petri dishes with HI-RGO (bottom inset of Fig. 3a ). This graphitic lining allowed the glassware to use HF. Finally, we note that most substrates used in our work had smooth surfaces (PET, metal foils). However, we have also tried GO coating on materials with rough surfaces such as, for example, conventional bricks. Despite brick’s highly porous structure, VC-RGO films exhibited excellent barrier properties, too ( Supplementary Fig. 4 and Supplementary Note 3 ). Furthermore, adhesion of RGO films to metal surfaces is found to be weaker than to plastic ones. This makes the protective coatings of metals more prone to mechanical scratching and peeling off. To overcome this problem, we have mixed a GO solution with polyvinyl alcohol (PVA) and used the binary solution to make GO-PVA films in the same manner as described in the methods. The resulting dry composites contained 30±10% of PVA. After their chemical reduction, the coatings exhibited practically the same barrier properties as without PVA but with much improved adhesion and mechanical characteristics ( Supplementary Fig. 5 and Supplementary Note 4 ). To explain the observed barrier properties of RGO, we recall that permeation through non-reduced GO laminates occurs via a network of graphene capillaries filled with one or two monolayers of water [5] , [6] . The capillaries have a width varying from 0.7 to 1.3 nm, depending on humidity. After chemical or thermal reduction, these capillaries collapse, and the interlayer separation decreases to only ≈0.36 nm, which is close to the interlayer separation in graphite [3] (see Fig. 3b ). This means that there is no space left for helium, water and other molecules to permeate between graphene sheets, and the only diffusion path remaining after the reduction is through structural defects. The crystallographic quality of reduced laminates can generally be judged by their X-ray diffraction peaks. Figure 3b shows that HI-RGO exhibits the sharpest peak indicating the highest degree of graphitization [3] , [27] . VC-RGO has a broader X-ray peak ( Fig. 3b ) but nonetheless shows barrier properties similar to those of HI-RGO. The only difference noticed between HI- and VC-RGO membranes was in their barrier properties with respect to moisture (see Fig. 1b ). The remnant H 2 O leakage for VC-RGO can be attributed to difficulties in reducing the membranes over their entire thickness by using VC that has larger and less mobile molecules than HI. However, approximately the same quality of graphitization for VC- and T-RGO films ( Fig. 3b ) indicates that factors other than the interlayer distance are important. We believe that the critical difference lies in the amount of structural defects formed during the reduction process. Indeed, it is known that during thermal reduction of GO, oxygen-containing functional groups are removed together with carbon atoms from graphene planes, which results in release of CO and CO 2 gases [3] , [23] . They have to escape from the interior and, therefore, can delaminate and damage the layered structure ( Supplementary Fig. 1 and Supplementary Note 1 ). On the contrary, chemical reduction by using HI and VC is much gentler, and most of the functional groups attached to graphene sheets react with the reducing agents releasing water instead of gases [3] , [23] , which can move along capillaries until they completely close behind [5] , [6] . As a result, our chemically reduced GO is less damaged and retains a better structural order (see Supplementary Note 1 ). In conclusion, chemically reduced GO films (especially, using HI) exhibit exceptional barrier properties with respect to all tested gases, liquids, salts and acids, with no detectable permeation. Although our accuracy with respect to moisture is limited to ≈10 −2 g m −2 per day, the known structural properties of HI-RGO allow us to expect that the moisture transmission should be similar to that for He and, therefore, would meet the stringiest industry requirements for flexible moisture barriers. The demonstrated films can be considered as thin graphitic linings, which can be produced on an industrial scale by solution processing. Taking into account that graphite is one of the most stable and chemically inert materials, this work opens a venue for many applications in which a barrier against moisture, oxygen and other gases and liquids is required and for the use in chemical and corrosion protection. The possibility to use the environment friendly reduction in ascorbic acid widens the scope of possible applications to sensitive areas including pharmaceuticals. Preparation of GO and RGO membranes and coatings Graphite oxide was prepared by the Hummers method [31] and then dispersed in water by sonication, which resulted in stable GO solutions [1] , [2] , [3] . The size of individual GO flakes varied from ~0.2–20 μm, and we did not find any notable size dependence in the barrier properties described above. We used two types of RGO samples: free-standing membranes and supported thin films on various substrates. The free-standing membranes were fabricated by vacuum filtration as described in refs 5 , 6 and had thickness d from 0.5 to 5 μm. The supported films were prepared by rod-coating [32] or spray-coating on top of 12-μm-thick PET films, metal foils and oxidized silicon wafers. Thermal reduction was carried out at 300 °C for 4 h in a hydrogen–argon mixture. HI reduction [25] , [27] was carried out by exposing GO films to the acid vapour at 90 °C. The exposure time varied from 5 to 30 min, depending on d . Then, samples were repeatedly rinsed with ethanol to remove residual HI. For VC reduction [26] , [28] , GO films were immersed in water solution of VC (30 g l −1 ) for 1 h at 90 °C. Optical and AFM characterization of HI-RGO on PET To characterize RGO films on PET, we have used scanning electron microscopy, atomic force microscopy (AFM) and optical absorption spectroscopy. Supplementary Fig. 2 shows an absorption spectrum for a 30-nm-thick film of HI-RGO. For the visible spectrum the transmittance varies from ≈30 to 40%. The thickness of RGO coatings was measured using a Veeco Dimension 3100 AFM in the tapping mode under ambient conditions. The inset of Supplementary Fig. 2 shows a representative AFM image for a 30-nm-thick HI-RGO on PET. Permeability measurements Permeation properties of the various RGO films were measured using several techniques that were described in detail previously [5] , [6] . In brief, for vapour permeation measurements, free-standing membranes and RGO-on-PET films were glued to a Cu foil with an opening of 2-cm diameter. The foil was clamped between two nitrile rubber O-rings sealing a metal container [5] . Permeability was measured by monitoring the weight loss of the container that was filled with water and other liquids inside a glovebox [5] . In gas permeation experiments [5] , GO-on-PET films were placed between two standard rubber gaskets and pressurized from one side to up to 1 bar. Gas permeation was monitored on the opposite (vacuum) side by using mass spectrometry. We used INFICON UL200 that allowed the detection of helium and hydrogen. Evaluating permeability from weight loss experiments Permeability P was calculated from our weight loss measurements as P = Q × d / A × Δ P , where Q is the weight loss rate, d the thickness of a membrane, A its area and Δ P the differential pressure of water vapour across the membrane. Moisture permeation experiments were carried out in a glove box with a negligible water vapour (<0.5 p.p.m.) so that Δ P was the partial pressure of water vapour at room temperature, that is,~2,300 Pa. How to cite this article: Su, Y. et al. Impermeable barrier films and protective coatings based on reduced graphene oxide. Nat. Commun. 5:4843 doi: 10.1038/ncomms5843 (2014).